Intrinsic electrical conductivity of nanostructured metal-organic polymer chains One-dimensional conductive polymers are attractive materials because of their potential in flexible and transparent electronics. Despite years of research, on the macro- and nano-scale, structural disorder represents the major hurdle in achieving high conductivities. Here we report measurements of highly ordered metal-organic nanoribbons, whose intrinsic (defect-free) conductivity is found to be 10 4 S m −1 , three orders of magnitude higher than that of our macroscopic crystals. This magnitude is preserved for distances as large as 300 nm. Above this length, the presence of structural defects (~ 0.5%) gives rise to an inter-fibre-mediated charge transport similar to that of macroscopic crystals. We provide the first direct experimental evidence of the gapless electronic structure predicted for these compounds. Our results postulate metal-organic molecular wires as good metallic interconnectors in nanodevices. Among other nanostructures, one-dimensional (1D) materials have given rise to great expectations because of their unique electrical transport properties as well as their potential utility in the emerging technology of transparent and flexible electronics [1] , [2] , [3] . For more than three decades, conjugated organic polymers were positioned as the best candidates for these purposes and they were extensively studied both at macro- and nano-scale [4] , [5] , [6] , [7] , [8] , [9] . Although remarkable improvement in their processability was achieved, the charge transport mechanisms and the limited conductivity found in fibres of organic polymers are still a matter of discussion [10] ; they show features typical of disordered materials where charge transport is described in terms of metallic islands surrounded by disordered regions that act as barriers. In the 1990s, this issue seemed to be resolved with the appearance of carbon nanotubes, purely carbon-based crystalline cylinders that exhibited unprecedented high conductivities [11] . Although the first reports showed promising results [12] , [13] , considerable effort was required to understand the tremendous influence of atomic scale defects on their conductivity [14] . Up to now, the lack of a cheap and massive procedure for the production of tubes with controlled chirality and low defect content has hindered their applicability. More recently, nanostructures based on metal-organic compounds [15] have been proposed as a viable and promising alternative [16] , [17] , [18] , [19] . These compounds allow the rational design of materials by self-assembly of selected building blocks [20] , [21] , [22] . However, the conductivities [17] reported so far for nanostructures and layered materials of metal-organic compounds are limited, as in organic polymers, by structural disorder. Therefore, the challenge of overcoming low conductivities and clarifying charge transport mechanisms relies on the production of well-ordered nanostructures and the ability to access their electrical properties below the length where disorder has a relevant role. In this work, we report the production of highly ordered nanoribbons where we are able to simultaneously achieve these two milestones. To this aim, we focus on the 1D MMX metal-organic polymer [Pt 2 ( dta ) 4 I] n formed by two simple moieties: a dimetallic subunit with two platinum centres connected by four bridging acetate ligands and an iodine atom bridging the dimetallic units. By direct sublimation of monocrystals of [Pt 2 ( dta ) 4 I] n on SiO 2 /Si supports, we form nanoribbons with a high degree of structural perfection. Each nanoribbon is composed of thousands of parallel MMX chains of ~0.8 nm diameter interacting by weak Van der Waals forces [23] . While the interatomic electron density along the chain is predicted to be high [16] , [24] , in the transversal direction, the electron density between chains is almost zero. This anisotropy gives rise to an extreme difference between the longitudinal (along the nanoribbon axis) and transversal electrical conductivities. The nanoribbons prepared in this way are characterized by conductive atomic force microscopy (CAFM). The small contact area characteristic of CAFM, along with the high electrical anisotropy of the material, reduces the paths of the current from thousands of chains to ~ 10. Plots of resistance versus length allow the intrinsic conductivity as well as the distance between defects, which dramatically influence charge transport, to be estimated. These are found to be 10 4 S m −1 and ~ 200 nm, respectively. Direct evidence of their inherent metallic character is also found, in good agreement with theoretical predictions [16] , [24] . When the electrical conduction properties of the nanoribbons are compared with those of the original crystals sublimated to prepare the nanorribons (with dimensions in the range of 10–300 μm), we obtain a significant improvement of three to four orders of magnitude. Interestingly, the electrical resistance of the conventional crystals scales linearly with the length of the crystal, in contrast with the exponential dependence observed for nanoribbons. The relationship between nano- and macro-scale properties is rationalized in terms of effective medium theory, showing that the inter-fibre transport is the limiting process in the crystals while transport along the polymeric chains dominates in the nanoribbons. 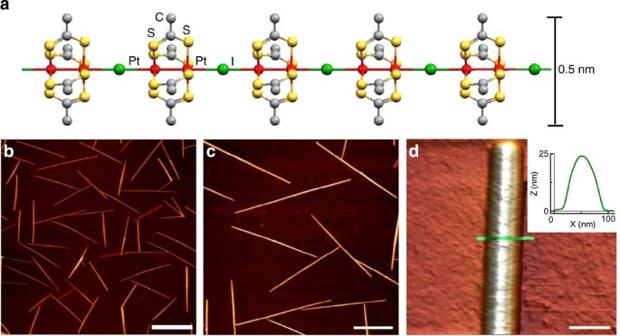Figure 1: Growth of nanoribbons with high degree of structural perfection by crystal sublimation. (a) Structure of a [Pt2(dta)4I]n(dta=dithioacetato) single fibre. (b,c,d) AFM images of nanoribbons on a SiO2substrate where the straightness and height homogeneity can be appreciated. The inset indis a profile acquired on the green line of the corresponding image, where the cross-section of the ribbons can be determined. Typical dimensions of the nanoribbons are 10 μm × 100 nm × 20 nm. Scale bars, 8, 4 and 0.1 μm (forb,candd, respectively). Electrical transport in nanoribbons Figure 1a provides a schematic representation of a single chain of [Pt 2 ( dta ) 4 I] n . The crystals were synthesized and characterized as described in Bellitto et al . [23] The nanoribbons were prepared by sublimating these crystals under high vacuum conditions on SiO 2 (300 nm)/Si(100) substrates previously treated with oxygen plasma (details can be found in the Methods section and Supplementary Figs S1 and S2 ). AFM images of the resulting nanoribbons are shown in Fig. 1b–d . Subsequent to nanoribbon growth, a macroscopic electrode was deposited by thermal evaporation of gold using a convenient stencil mask. The final result is a long gold electrode edge that partially covers a number of nanoribbons. The electrical resistance of the nanostructure was probed by CAFM [25] , [26] . 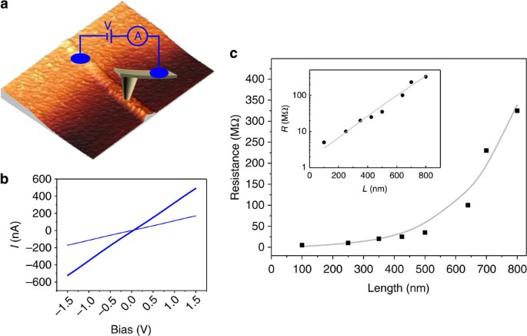Figure 2: Electrical characterisation of MMX nanoribbons by conductive AFM. (a) Scheme of the electronic circuit used to measure the current flowing through the nanoribbons, a metallized AFM tip is used as a mobile electrode. (b)I/Vcurves obtained at different distances between electrodes (lengths) for the same nanoribbon. Here it can be clearly seen that the linear behaviour is maintained for every point. Resistance is calculated as the inverse of the slope of these graphs. (c) Resistance versus length, in a linear scale, for the same nanoribbons as data depicted inb. The inset displays a semi log plot of the same experimental data. Black dots represent experimental measurements and grey line is a fit to Figure 2a shows a representative AFM image of a nanoribbon protruding from a gold electrode, and a scheme of the electrical circuit was used to characterize the ribbon. Figure 2c displays the electrical resistance R , as a function of the distance between electrodes L , obtained for a representative nanoribbon. The resistance displays an initial region where it barely depends on length followed by a rapid increase that can be fitted well to an exponential law. The current versus voltage ( I / V ) curves acquired for the nanoribbons and depicted in Fig. 2b show a linear dependence, and hence the resistance for each data point in Fig. 2c is independent of the bias voltage. Figure 1: Growth of nanoribbons with high degree of structural perfection by crystal sublimation. ( a ) Structure of a [Pt 2 ( dta ) 4 I] n ( dta =dithioacetato) single fibre. ( b , c , d ) AFM images of nanoribbons on a SiO 2 substrate where the straightness and height homogeneity can be appreciated. The inset in d is a profile acquired on the green line of the corresponding image, where the cross-section of the ribbons can be determined. Typical dimensions of the nanoribbons are 10 μm × 100 nm × 20 nm. Scale bars, 8, 4 and 0.1 μm (for b , c and d , respectively). Full size image Figure 2: Electrical characterisation of MMX nanoribbons by conductive AFM. ( a ) Scheme of the electronic circuit used to measure the current flowing through the nanoribbons, a metallized AFM tip is used as a mobile electrode. ( b ) I / V curves obtained at different distances between electrodes (lengths) for the same nanoribbon. Here it can be clearly seen that the linear behaviour is maintained for every point. Resistance is calculated as the inverse of the slope of these graphs. ( c ) Resistance versus length, in a linear scale, for the same nanoribbons as data depicted in b . The inset displays a semi log plot of the same experimental data. Black dots represent experimental measurements and grey line is a fit to Full size image The observed non-linear dependence of R(L) suggests that electron–defect interactions are the main source of resistance in these nanoribbons and can be explained with a simple model of polymeric chains connected in parallel. We assume that ρ 1D (intrinsic resistivity from now on) accounts for different contributions such as Landauer-type resistance, electron–phonon interaction and electron–electron interaction, but it does not consider the presence of disorder. We then assume a random configuration of defects that interrupt the current through a single molecular wire (we expect vacancies of either iodine atoms or dimetallic subunits [27] ). The probability P of molecular wire being continuous (defect-free) decays exponentially with the length L as P(L)=exp(−L/Λ) , where Λ is the mean distance between defects. Including an electrode–nanoribbon contact resistance R c , the electrical resistance can be written as: Because we perform superficial contacts, we consider that only the wires directly contacted by the AFM probe contribute to the electrical current. Because of the high electrical anisotropy of the nanoribbons, those in the second layer or outside the tip contact area will exhibit a much higher electrical resistance and can be safely neglected. The number of wires contacted by the AFM tip can be estimated using Hertz’s model, as explained in Welte et al . [16] and in the Supplementary Note 1 . The contact region has a circular shape with a typical diameter of ~12 nm. As the distance between chains is ~0.8 nm, according to X-ray data [23] , N 0 ~10–20. For all the measured nanoribbons, the experimental R ( L ) curves are fitted well by equation (1). Numerical fitting of the data shown in Fig. 2c leads to ρ 1D ≈0.1 MΩ nm −1 , Λ ≈212 nm and R c ≈ 2 MΩ. The exact values change for different nanoribbons, but the ranges are small (0.02< ρ 1D <0.1, 124< Λ <230 nm and 1< R c < 12 MΩ). The estimated density of defects c is 0.4–1% (see Supplementary Note 2 for details), implying that there is one defect every 80–210 nm in each polymeric chain. Ideally, if we could prepare defect-free crystals, their intrinsic three-dimensional (3D) conductivity would be σ 3D ≈2 × 10 4 S m −1 , higher than that reported for the best conjugated polymer nanofibres [10] . In the present nanoribbons, this intrinsic conductivity occurs for lengths as large as a few hundred nanometres. The I/V curves ( Fig. 2b ) show a clear linear dependence independently of the position at which the curve is measured, suggesting an inherent metallic character. Although this metallic behaviour has been predicted by density functional theory calculations [16] , [24] , it has not yet been observed experimentally. To corroborate this behaviour, we performed electrical transport measurements in a field effect transistor configuration (see Methods section and Supplementary Figs S3 and S4 ). The absence of gate-dependent resistance confirms the gapless band structure. The results were similar for both high (Au) and low (Ti) work function metals, ruling out injection or contact effects. Electrical transport in conventional crystals With the aim of a full characterization of the material, the measurements were extended to conventional (micro-scaled) monocrystals of the same compound with typical dimensions of 350 × 10 × 10 μm 3 . Measurements of several crystals, in four-probe configuration, gave longitudinal conductivity values of 10–80 S m −1 , three or four orders of magnitude lower than those obtained for the intrinsic value of the polymeric chains. In contrast with the exponential R(L) dependence of the nanoribbons, the electrical resistance of the crystal as a function of the length ( Fig. 3a ) showed a linear dependence. In addition, the curves showed a marked non-linear behaviour ( Fig. 3b ), clearly indicating a change in the electrical transport mechanism from the nanoribbons to the crystals. Two-terminal transversal conductivity measurements (perpendicular to the polymer chains axis) resulted in values of 10 −4 –10 −3 S m −1 , reflecting the very high electrical anisotropy in the electrical properties of these crystals. 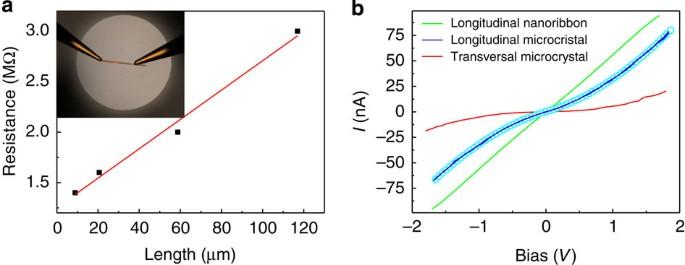Figure 3: Electrical characterisation of conventional MMX crystals. Comparison ofIVcurves for the nanoribbons and macrocrystals. (a) Resistance versus length curve acquired on a crystal with dimensions of 350 × 10 × 10 μm3, where, in contrast to the nanoribbons case, a linear behaviour is observed. The inset shows an optical microscopy image of a crystal contacted by two gold probes. (b) ExperimentalI/Vcurves obtained for nanoribbons (green), and crystals both for longitudinal transport (blue) and for transversal transport (red). The light blue empty circles show the fitting to theoretical Expression (2) of the main text. Figure 3: Electrical characterisation of conventional MMX crystals. Comparison of IV curves for the nanoribbons and macrocrystals. ( a ) Resistance versus length curve acquired on a crystal with dimensions of 350 × 10 × 10 μm 3 , where, in contrast to the nanoribbons case, a linear behaviour is observed. The inset shows an optical microscopy image of a crystal contacted by two gold probes. ( b ) Experimental I/V curves obtained for nanoribbons (green), and crystals both for longitudinal transport (blue) and for transversal transport (red). The light blue empty circles show the fitting to theoretical Expression (2) of the main text. Full size image Numerical simulations In crystals with lengths L >> Λ , all polymeric chains have at least one defect and, hence, transport perpendicular to the polymer chains becomes determinant. This regime dominates for microscopic samples. To study the transition between the L ≤ Λ and L >> Λ regimes, we performed extensive numerical simulations in an anisotropic 3D resistor model ( Supplementary Note 2 for details). These simulations support the R(L) dependences observed in both the nanoribbons and the crystals ( Fig. 4 ) and confirm that the regime observed in crystals can be understood using the Effective Medium Theory applied to anisotropic systems ( Supplementary Note 3 ) [28] , [29] , [30] . This theory relates effective conductivities, σ ||eff and eff , measured in macroscopic crystals, and intrinsic (free of defects) conductivities, σ ||int and int , measured using CAFM, where || and indicate the directions parallel and perpendicular to the polymeric chains, respectively. Considering that the only source of disorder is the chain-interrupting defect, we assume that eff = int . With such a limit, high anisotropy and small defect concentration, the effective conductivity decreases to the simple expression σ ||eff = eff 0.918/ c 2 independently of the sample size, as found experimentally. From this expression, we calculate that the defect densities for both crystals and nanoribbons are very similar (0.4%< c <1%), see Supplementary Fig. S5 . The simulations also disclose a crossover regime ( L ≈ Λ ), which matches the nanoscopic and microscopic regimes. Details about this crossover regime and a simple analytical fit to the numerical data are given in the Supplementary Note 4 and Supplementary Figs S6 and S7 . 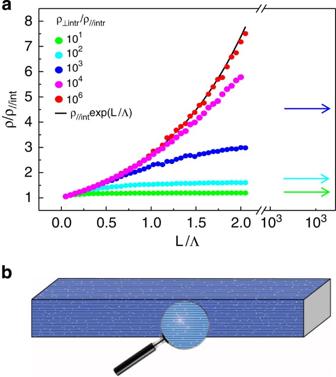Figure 4: Theoretical modelling, anisotropic and disorder media. (a) Normalized resistivity versus length of the sample (in units ofΛ) for different values of anisotropy as computed in the 3D resistor model. Black arrows correspond to the EMT result. All the transport regimes described in the main text are depicted in this graph; for small lengths, the resistivity (and resistance) depends exponentially on the sample length, and for larger lengths, it saturates to the value predicted by Effective Medium Theory. The figure also illustrates the importance of high anisotropy in the observation of the different regimes depending on the measured length scale. For the more anisotropic samples, the exponential dependence can be observed for larger lengths. (b) Schematic view of the structure of a MMX crystal showing the polymeric chains and a random distribution of defects (lighter regions). Figure 4: Theoretical modelling, anisotropic and disorder media. ( a ) Normalized resistivity versus length of the sample (in units of Λ ) for different values of anisotropy as computed in the 3D resistor model. Black arrows correspond to the EMT result. All the transport regimes described in the main text are depicted in this graph; for small lengths, the resistivity (and resistance) depends exponentially on the sample length, and for larger lengths, it saturates to the value predicted by Effective Medium Theory. The figure also illustrates the importance of high anisotropy in the observation of the different regimes depending on the measured length scale. For the more anisotropic samples, the exponential dependence can be observed for larger lengths. ( b ) Schematic view of the structure of a MMX crystal showing the polymeric chains and a random distribution of defects (lighter regions). Full size image The situation in which the charge transport mechanism at the nanoscale is completely different to the processes dominating charge transport at the macroscale has been previously observed in conjugated conducting polymers [31] . To clarify these mechanisms and their contributions, disorder should be reduced until the studied sizes are in a range where it can be ignored. For the case of organic polymers, this situation has been historically too difficult to reach, and charge transport mechanisms are still a matter of intense debate. The situation for metal-organic materials was analogous until now. To reverse this situation, we had to simultaneously achieve a high structural order and characterization at the nanometre scale. This was possible due to the excellent processability of these metal-organic polymers [27] , [32] , which show the exceptional feature of undergoing reversible depolymerization/repolymerization during sublimation, as well as the fine tuning of the parameters affecting the repolymerization process on the surface. Although the achieved characteristic length of 200 nm is already enough for many current devices, our on-going work focuses on increasing this distance further. Finally, in the case of quasi-1D systems, it is known that electron–electron interactions lead to phases that are different from conventional Fermi liquids, such as Luttinger Liquids or Wigner Crystals. Some experimental studies on polymer nanofibres and nanotubes have already shown features characteristic of 1D systems [10] . In our crystals, while fits to conventional hopping models show a poorer agreement, the I ( V ) curves in the parallel direction can be fitted by [33] : Where Γ is the Gamma function, V is the bias voltage, T is the temperature (300 K) and K B is the Boltzman constant, suggesting a 1D electronic behaviour with a single band crossing the Fermi level. The fitting values are I 0 =0.12 nA, α =0.937 (the critical exponent for the density of states) and G N =0.185 × 10 −7 S, which represents a parallel conductance. Unfortunately, temperature-dependent measurements in these samples are challenging and difficult to interpret due to a crystal structural transition near room temperature [34] . A complete identification of such 1D behaviour would require temperature-dependent studies on nanoribbons, and work in this respect is currently underway. In summary, we demonstrate that highly ordered platinum-based MMX 1D structures are able to transport electrical carriers more efficiently than 1D conjugated organic polymers. By taking advantage of the self-assembly capability of this compound, we have been able to prepare, in an easy way, 1D structures, with low defect content (0.4%< c< 1%), that present an intrinsic conductivity of 10 4 S m −1 . Also, owing to the low structural disorder, we have been able to experimentally confirm the predicted gapless band structure of this material. This work constitutes a unique case of study of the influence of a small concentration of defects in metal-organic systems with high electrical anisotropy. The ideas and methodology presented here are expandable to other similar polymeric compounds and can be applied to the study of the emerging nanostructured metal-organic polymer family [32] . Crystal sublimation and structural characterization of ribbons Well-ordered 1D nanoribbons on SiO 2 surfaces were isolated by direct sublimation from monocrystals of [Pt 2 I(S 2 CCH 3 ) 4 ] n . The approach involved the deposition from the vapour phase on a substrate of species obtained upon sublimation of [Pt 2 I(S 2 CCH 3 ) 4 ] n crystals under high vacuum conditions, and their self-organisation on the host surface. In a vacuum chamber, with a base pressure of 1 × 10 −6 mbar, [Pt 2 I(S 2 CCH 3 ) 4 ] n crystals were gradually annealed up to 180 °C, and then heated at this temperature for 1.5 h, whereas the SiO 2 substrates were kept at 40 °C to allow a suitable diffusion of the landing species. It was observed that maintaining the substrate temperature once the sublimation process was completed (diffusion time ca. 15 min), as well as adjusting the slow and gradual deposition of material, had an important role in the formation of well-ordered and homogeneous nanostructures on the substrate. Under these conditions, a high density of straight, long and homogenous ribbons with typical cross-sections of 20 × 100 nm 2 and up to 10 μm in length were obtained (see for example, Supplementary Fig. S1 for more information). The AFM morphological characterization was performed with Olympus-type cantilevers with 0.75 N m −1 nominal stiffness and resonance frequencies of 70 kHz. The images were acquired with a Nanotec Electrónica system working in the amplitude modulation mode to avoid damaging the samples. The data were acquired and processed using WSxM software [35] . Conductive AFM characterisation of the nanoribbons Commercial gold-coated Budget Sensors cantilevers having 3 N m −1 nominal force constant and resonance frequencies of about 75 kHz were used in the experiments. Tip radius is 25/30 nm according to the data provided by the manufacturer (Budget Sensors: Multi75GB-G). Electrical characterization of the MMX nanoribbons was performed by conductance AFM at room temperature in ambient air conditions. To this end, a macroscopic gold electrode was evaporated on previously prepared samples, resulting in a number of nanoribbons partially covered by this fixed electrode. With a metallic AFM tip used as a second mobile electrode, the uncovered parts of the nanoribbons were contacted, measuring the current versus voltage characteristics ( I–V ) as a function of the distance between the tip and the fixed electrode. From the I–V plots, the resistance versus length curve R(L) was determined along the nanoribbon by fitting a straight line to the data around zero volts. The experimental setup enabled increasing the loading force applied by the mobile electrode to the nanoribbon while the current versus voltage ( I–V ) characteristics were measured, until an optimum contact resistance was reached. In this way, simultaneous force-distance F ( z ) and current-distance I ( z ) curves were obtained ( z being the piezoelectric displacement along the perpendicular direction to the sample surface). The maximal current was measured for an applied force of 50 nN. The same force was used for all the measurements reported in the manuscript. The dependence of the electrical resistance of the nanoribbons as a function of their length is characterized by CAFM. The experimental procedure is as follows: (i) the metallized AFM tip is brought into mechanical and electrical contact with the sample; (ii) a bias ramp is applied to the tip while the current is monitored; and (iii) the tip is withdrawn and moved to the next point. Electrical characterisation of the nanoribbons in a field-effect configuration Samples for electrical characterisation in FET configuration were prepared by metal evaporation with a stencil mask on SiO 2 /Si/metal substrates with previously deposited nanoribbons ( Supplementary Fig. S3 ). Gold and titanium electrodes were used. AFM inspection of the substrate revealed nanoribbons that contacted both fixed electrodes, and the distance between electrodes was between 0.4 and 1.5 μm. The variation of the current versus bias applied across the nanoribbons as a function of the back-gate voltage was measured ( Supplementary Fig. S4 ). Measurements were performed both in an ambient and an argon atmosphere. No difference was detected. Additional details on crystal sublimation conditions, electrical transport measurements, sample preparation, calculation of contact area of the AFM tip with the ribbon and theoretical modelling can be found in Supplementary Figs S4–S7 and Supplementary Note 1–4 . How to cite this article: Hermosa, C. et al . Intrinsic electrical conductivity of nanostructured metal-organic polymer chains. Nat. Commun. 4:1709 doi: 10.1038/ncomms2696 (2013).